Real-space observation of spin-split molecular orbitals of adsorbed single-molecule magnets A key challenge in the field of molecular spintronics, and for the design of single-molecule magnet-based devices in particular, is the understanding and control of the molecular coupling at the electrode interfaces. It was demonstrated for the field of molecular electronics that the characterization of the molecule-metal-interface requires the precise knowledge of the atomic environment as well as the molecular orbitals being involved in electron transport. To extend the field of molecular electronics towards molecular spintronics, it is of utmost importance to resolve the spin character of molecular orbitals interacting with ferromagnetic leads. Here we present first direct real-space images of spin-split molecular orbitals of a single-molecule magnet adsorbed on a ferromagnetic nanostructure. Moreover, we are able to determine quantitatively the magnitude of the spin-splitting as well as the charge state of the adsorbed molecule. Single-molecule magnets (SMM) exhibit new properties such as electric control of molecular spin states [1] , remarkably high blocking temperatures, hysteresis [2] , quantum tunnelling of magnetization [3] , [4] , and tunable coupling to magnetic substrates [5] . Recently, the realization of novel devices, such as multiple-field-effect nanotransistors [6] or supramolecular spin valves [7] has been reported, demonstrating the potential of SMMs for technological applications, in particular spintronics [8] and quantum computing [9] , [10] . Further progress in the field requires a detailed understanding of structural properties and magnetic interactions of an individual SMM in contact with a ferromagnetic electrode in an atomically well-defined environment. We select bis(phthalocyaninato)terbium(III) (TbPc 2 ) as a model-type system because of its high blocking temperature ( T B ~30–50 K) [11] , [12] , its comparably small size and its high stability that allows for thermal deposition in ultrahigh vacuum environments. The structure of a TbPc 2 molecule is depicted in Fig. 1a . It consists of a Tb ion sandwiched between two phthalocyanine (Pc) rings. The upper Pc ring is staggered by 45° with respect to the lower plane [13] , but it requires little energy to modify this twisting angle [14] . Neutral TbPc 2 ([TbPc 2 ] 0 ) contains two spin systems: a central J =6 Ising-type high-spin system arising from the Tb 4f-electrons, and a peripheric S =1/2 π -radical delocalized over the two Pc ligands [15] . In neutral [TbPc 2 ] 0 , the highest occupied molecular orbital (HOMO), which is delocalized over both Pc rings [15] , is therefore just singly occupied. With spin-polarized scanning tunnelling microscopy (SP-STM), this ligand spin should be observable as follows: as the singly occupied molecular orbital of [TbPc 2 ] 0 is also the lowest unoccupied molecular orbital (LUMO) [16] , it should be visible both below as well as above the Fermi level. Because of the Pauli exclusion principle, these orbitals have opposite spin character ( Fig. 1a ). Komeda et al . [1] have shown that the ligand spin of TbPc 2 in molecular assemblies can be switched on and off through the modification of the twisting angle. On the other hand, experimental and theoretical studies on phthalocyanine molecules show that the charge and spin state of single molecules may be altered on adsorption on surfaces [17] . Therefore, both the twisting and the adsorption-induced charging of [TbPc 2 ] 0 molecules can cause a quenching of the ligand spin ( Fig. 1b ). To unambiguously identify the spin state of an adsorbed TbPc 2 molecule, a direct spin-resolved study of specific ligand orbitals is required. Spin-resolved investigations of simple Pc molecules on ferromagnetic substrates by SP-STM [18] , [19] showed that the spin structure of molecule–substrate hybrid systems can indeed be mapped with high spatial and energy resolution [20] , [21] . 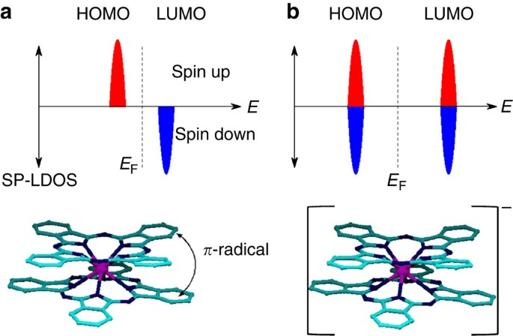Figure 1: Schematic spin-resolved states of TbPc2close to the Fermi level (EF). (a) Neutral [TbPc2]0: as the HOMO is singly occupied by aπ-radical, the entire orbital is split into an occupied state below and an unoccupied state above the Fermi energy. Because of the Pauli exclusion principle, their spins are of opposite sign. (b) Negatively charged [TbPc2]−: theπ-radical is quenched by reduction with the additional electron. Consequently, there is no spin-split state across the Fermi level16. Figure 1: Schematic spin-resolved states of TbPc 2 close to the Fermi level ( E F ). ( a ) Neutral [TbPc 2 ] 0 : as the HOMO is singly occupied by a π -radical, the entire orbital is split into an occupied state below and an unoccupied state above the Fermi energy. Because of the Pauli exclusion principle, their spins are of opposite sign. ( b ) Negatively charged [TbPc 2 ] − : the π -radical is quenched by reduction with the additional electron. Consequently, there is no spin-split state across the Fermi level [16] . Full size image Here we directly observe the spin-splitting of molecular orbitals of TbPc 2 molecules deposited on a ferromagnetic cobalt support. The spin polarization of individual molecules is mapped on a sub-molecular scale by low-temperature SP-STM, and the spin-splitting of the LUMO is determined quantitatively. 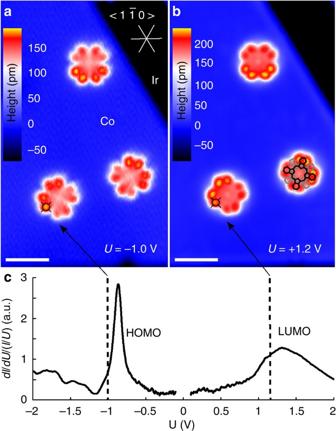Figure 2: Spin-averaged STM and point spectroscopy data of TbPc2on cobalt islands on Ir. (a,b) Spin-averaged STM topographs of three TbPc2molecules on cobalt islands on Ir. The bias voltage is chosen to image either the HOMO (a) or the LUMO (b). Inb, one molecule is overlaid with a model of TbPc2with the upper Pc ring drawn in black and the lower one in grey. White scale bars correspond to 2 nm. (c) Spin-averaged differential tunnelling spectroscopy, normalized by dividing byI/U. Electronic structure and adsorption geometry of TbPc 2 Figure 2a,b presents STM topographs of a Co nanostructure on Ir(111) together with three TbPc 2 molecules exhibiting three distinct orientations. The individual molecules are well separated from one another, in contrast to a similar preparation of these molecules on a Au(111) surface [1] , where the TbPc 2 molecules assemble into islands. The comparison of molecular adsorption on the two different substrates indicates that molecule–substrate interactions are much stronger when TbPc 2 molecules are in contact with Co as compared with Au, where molecule–molecule interactions dominate. This argument is further strengthened by the observed molecular orientation discussed in Supplementary Fig. S1 and Supplementary Methods . Figure 2: Spin-averaged STM and point spectroscopy data of TbPc 2 on cobalt islands on Ir. ( a , b ) Spin-averaged STM topographs of three TbPc 2 molecules on cobalt islands on Ir. The bias voltage is chosen to image either the HOMO ( a ) or the LUMO ( b ). In b , one molecule is overlaid with a model of TbPc 2 with the upper Pc ring drawn in black and the lower one in grey. White scale bars correspond to 2 nm. ( c ) Spin-averaged differential tunnelling spectroscopy, normalized by dividing by I / U . Full size image The spin-averaged electronic structure of TbPc 2 is investigated by point spectroscopy above the ligand. The spin-averaged normalized differential tunnelling conductance (d I /d U )/( I / U ) ( Fig. 2c ) shows two pronounced peaks at U =−0.9 V and U =+1.3 V. These features are attributed to the HOMO and the LUMO, respectively. The spatial distribution of these states is imaged in the respective topographs in Fig. 2a,b and shows an eight-lobe structure for both HOMO and LUMO. This particular appearance is characteristic for π -orbitals of phthalocyanine molecules only weakly interacting with the surface [22] . The fact that we observe this eight-lobe structure for the TbPc 2 molecules as well indicates that we are imaging the molecular orbital contribution originating from the upper Pc ring, which is only weakly electronically interacting with the Co support. The appearance of an eight-lobe structure is expected for both a neutral [TbPc2] 0 (with the ligand spin still present) as well as for a negatively charged [TbPc 2 ] − molecule (with the ligand spin quenched by the reduction with the additional electron) [16] . Therefore, spin-averaged measurements cannot distinguish between the charged and the neutral state of adsorbed TbPc 2 . Moreover, spin-averaged measurements cannot determine the spin state of the frontier orbitals. To address the spin character of these orbitals, SP-STM data is collected. 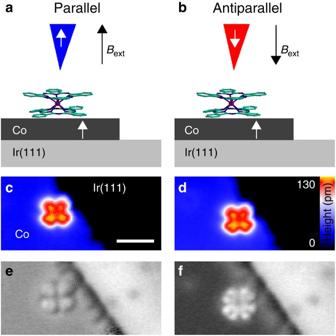Figure 3: Schematic diagram of SP-STM experiments as performed here. To obtain spin sensitivity, the magnetization direction of the tip is aligned either parallel (blue/dark) or antiparallel (red/light grey) by applying an external magnetic field ofB=±1 T. The Co nanostructure is a hard magnet with a magnetization that does not rotate with the field applied here. Because of the tunnel magnetoresistance effect, the tunnelling current depends on the relative alignment of tip and sample magnetization directions, thereby giving spin sensitivity. To isolate the spin-polarized component, signals from measurements with parallel (a) and antiparallel (b) alignments of tip and sample magnetization are subtracted from each other. (c–f) Example of a spin-resolved measurement: SP-STM topographs (c, parallel;d, antiparallel) and spin-resolved maps of differential conductance (e, parallel;f, antiparallel) taken atU=−0.5 V. The white scale bar corresponds to 2 nm. The topographs (c,d) show little difference, the maps of spin-resolved differential conductance (e,f) do: the Co island appears brighter for parallel alignment of tip and sample magnetization. Not only the Co island, but also the TbPc2molecule shows magnetic contrast, that is, an eight-lobe structure for antiparallel and a cross-shape for parallel alignment. Spin-resolved investigation of TbPc 2 molecules Figure 3a,b presents a scheme of SP-STM, as it is employed here: to gain spin sensitivity, a tungsten tip is coated with a ferromagnetic material (iron). TbPc 2 molecules are deposited on a ferromagnetic cobalt nanostructure exhibiting a magnetization along the surface normal. To probe the two different spin channels (parallel and antiparallel), the tip magnetization (soft magnet) is aligned out of plane, either parallel or antiparallel to the magnetization of the cobalt nanostructure, by applying an external magnetic field of ±1 Tesla. Because of their high coercivity, the Co nanostructures act as hard magnets; therefore, their magnetization does not rotate with the external field applied here. The resulting parallel ( Fig. 3a ) and antiparallel (b) configurations give different tunnelling currents. The difference of these two spin channels is a measure of the spin polarization of the sample [19] . Figure 3: Schematic diagram of SP-STM experiments as performed here. To obtain spin sensitivity, the magnetization direction of the tip is aligned either parallel (blue/dark) or antiparallel (red/light grey) by applying an external magnetic field of B =±1 T. The Co nanostructure is a hard magnet with a magnetization that does not rotate with the field applied here. Because of the tunnel magnetoresistance effect, the tunnelling current depends on the relative alignment of tip and sample magnetization directions, thereby giving spin sensitivity. To isolate the spin-polarized component, signals from measurements with parallel ( a ) and antiparallel ( b ) alignments of tip and sample magnetization are subtracted from each other. ( c – f ) Example of a spin-resolved measurement: SP-STM topographs ( c , parallel; d , antiparallel) and spin-resolved maps of differential conductance ( e , parallel; f , antiparallel) taken at U =−0.5 V. The white scale bar corresponds to 2 nm. The topographs ( c , d ) show little difference, the maps of spin-resolved differential conductance ( e , f ) do: the Co island appears brighter for parallel alignment of tip and sample magnetization. Not only the Co island, but also the TbPc 2 molecule shows magnetic contrast, that is, an eight-lobe structure for antiparallel and a cross-shape for parallel alignment. Full size image First, magnetic contrast is established using the ferromagnetic Co islands as a reference ( Fig. 3c–f ): At U =−0.5 V, Co islands appear bright, when their magnetization direction is aligned parallel to the tip magnetization direction, and dark in the antiparallel case [23] . TbPc 2 molecules adsorbed on the ferromagnetic Co islands show a strong spin-dependent contrast as well: a clear eight-lobe state for an antiparallel and a cross-like appearance for a parallel alignment of tip and sample magnetization directions. Spin-splitting of the LUMO After spin contrast has been established, we focus on the analysis of the spin character of the LUMO. 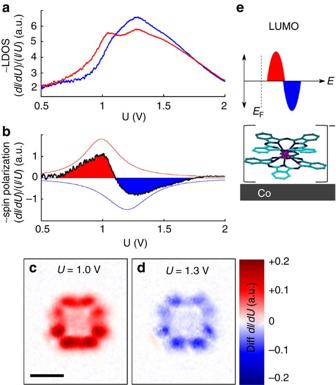Figure 4: Spin-resolved STM and point spectroscopy data of the LUMO. (a) Spin-resolved point-mode spectroscopy of TbPc2. Blue (dark), parallel alignment of tip and sample magnetization direction; red (light grey), antiparallel. (b) Difference of the spectroscopic curves of the antiparallel and parallel case from (a), providing a measure of the spin polarization. The area of blue (dark) and red (light grey) parts are equal, indicating that there is no net magnetization. Smooth red and blue curve: fit by two Lorentzian functions. (c,d) Differences of maps of spin-resolved differential tunnelling conductance for (c)U=+1.0 V and (d)U=+1.3 V, providing maps of the spin polarization of the molecular orbitals at the given voltages. Both orbitals show the same spatial distribution, but have opposite spin polarization. The black scale bar corresponds to 1 nm. (e) Schematic of the electronic structure of TbPc2adsorbed on a cobalt nanostructure, depicted according toFig. 1. Figure 4 summarizes the experimental findings: the point spectroscopy mode data ( Fig. 4a ) show that the broad feature with a maximum at U =+1.3 V, which we assigned to the LUMO in the spin-averaged measurements ( Fig. 2c ), contains two spectroscopic features: the first feature at U =+1.0 V is clearly visible only if tip and sample magnetizations are aligned antiparallel (in the following referred to as LUMO ap ), whereas the second feature at U =+1.2 V is more pronounced if tip and sample magnetizations are aligned parallel (LUMO p ). Figure 4b depicts the difference of spin-resolved normalized differential tunnelling conductance for antiparallel and parallel alignment, which is a measure of the spin polarization of LUMO ap and LUMO p . Clearly, LUMO ap is of opposite spin character compared with LUMO p . Their exact energetic positions are determined by fitting two Lorentzian functions. The areas below the "antiparallel'' and the "parallel'' LUMO features are equal, indicating that the total spin polarization of the entire LUMO is zero. After determining the spin character of these states in point spectroscopy mode, we map the spatial distribution of both states in the spin-split LUMO. To do this, we perform constant height-mode measurements. To avoid any topographic effects in SP-STM data [24] , the tip is stabilized above the non-magnetic Ir substrate, which results in the same tip-sample distance for both parallel and antiparallel alignment of the tip and the Co-island magnetization direction. The difference between the antiparallel and parallel case yields information about the spatial distribution of the molecular spin polarization ( Fig. 4c,d ): for U =+1.0 V, it is positive, and negative for U =+1.3 V, consistent with the point spectroscopy data. More importantly, both orbitals are clearly of eight-lobe character. This proves that both features originate from the LUMO π -orbital. The fact that LUMO ap and LUMO p have an identical spatial distribution with opposite spin character allows us to unambiguously attribute the two spectral features in the different spin channels to the same molecular orbital, that is, we spatially and energetically resolve the spin-splitting of the LUMO. The magnitude of the spin-splitting of the LUMO amounts to As shown above, the total spin polarization of the LUMO is zero, thereby excluding the presence of a radical spin in the LUMO ( Fig. 4e ). Figure 4: Spin-resolved STM and point spectroscopy data of the LUMO. ( a ) Spin-resolved point-mode spectroscopy of TbPc 2 . Blue (dark), parallel alignment of tip and sample magnetization direction; red (light grey), antiparallel. ( b ) Difference of the spectroscopic curves of the antiparallel and parallel case from ( a ), providing a measure of the spin polarization. The area of blue (dark) and red (light grey) parts are equal, indicating that there is no net magnetization. Smooth red and blue curve: fit by two Lorentzian functions. ( c , d ) Differences of maps of spin-resolved differential tunnelling conductance for ( c ) U =+1.0 V and ( d ) U =+1.3 V, providing maps of the spin polarization of the molecular orbitals at the given voltages. Both orbitals show the same spatial distribution, but have opposite spin polarization. The black scale bar corresponds to 1 nm. ( e ) Schematic of the electronic structure of TbPc 2 adsorbed on a cobalt nanostructure, depicted according to Fig. 1 . Full size image In this experiment ( T =6 K), we do not observe any spin polarization directly arising from the central Tb atom. Moreover, the second spin system of [TbPc 2 ] 0 , the S =1/2 ligand spin, is not present here, as shown above. Nevertheless, there is a spin-split on the LUMO, whose clear eight-lobe structure closely resembles a pristine molecular orbital. The spin-splitting of the LUMO can either arise owing to coupling to the ferromagnetic Co support, or be mediated by the Tb ion. Because the 4f-electrons of the Tb ion are highly localized, a direct coupling of the Tb ion to the Co support is unlikely (recent studies assume a superexchange coupling mediated via the Pc ligand [5] ). Additionally, calculations by Vitali et al . [16] do not show a spin-splitting for the ligands for free and negatively charged TbPc 2 and for molecules in contact with Cu(111) surfaces. Therefore, we attribute the spin-splitting of the LUMO to a direct magnetic coupling of the Co support to both Pc rings. In conclusion, we have spatially and energetically resolved the highest occupied and the lowest unoccupied molecular orbital. Moreover, we have mapped the spatial distribution of both spin-components of a spin-split molecular orbital on a sub-molecular level. The spin-splitting has been determined to be on the order of 210 meV. Furthermore, we conclude that the ligand spin is quenched on the upper ring upon adsorption of TbPc 2 molecules on the Co nanostructures. As in ref. 1 , the Tb magnetic moment was not directly accessible, raising the importance of the ligand spin system for applications in spintronic devices. The observation of a spin-split molecular orbital even in the absence of a radical spin on the ligand is a crucial result of our experimental study. Experimental set-up All measurements are performed with a home-built SP-STM [25] under ultrahigh vacuum conditions at a temperature of 6 K. Magnetic fields are applied parallel or antiparallel to the surface normal. Spin-sensitive probe tips (W tips coated with ~50 monolayers of Fe) and ferromagnetic cobalt nanostructures on an Ir(111) substrate are prepared in vacuo , according to the procedure described in ref. 23 . Sample preparation TbPc 2 molecules are synthesized, as described before [13] , degassed in vacuo at ~300 °C for several days, and sublimated in situ from a ceramic Knudsen cell [26] held at ~400 °C directly onto the sample kept at room temperature. Following molecule deposition, the sample is directly transferred into the SP-STM system and cooled down to measurement temperature. Supplementary Fig. S2 proves that the molecules remain intact on deposition. Additional information on the molecular adsorption, discussing molecule–substrate interaction and twisting angle, can be found in the supplement. Data acquisition The differential conductance is recorded using lock-in technique with parameters given below. Point spectra are normalized by dividing by I / U . STM and point spectroscopy parameters: Fig. 2a,b : I =100 pA Fig. 2c : U stab =+2 V, I stab =1 nA, U mod =50 mV rms , f mod =6777 Hz Fig. 3 : I =1 nA, U mod =50 mV rms , f mod =6777 Hz, B =±1 T Fig. 4a,b : Curves for both spin channels have been averaged over 32 spectra taken over all 8 lobes. U stab =+2 V, I stab =1 nA, U mod =10 mV rms , f mod =6777 Hz, B =±1 T Fig. 4c,d : I stab =1 nA, Δ z stab =−4.5 Å, U mod =50 mV rms , f mod =6777 Hz, B =±1 T. How to cite this article: Schwöbel, J. et al . Real-space observation of spin-split molecular orbitals of adsorbed single-molecule magnets. Nat. Commun. 3:953 doi: 10.1038/ncomms1953 (2012).